Organogenesis relies on SoxC transcription factors for the survival of neural and mesenchymal progenitors During organogenesis, neural and mesenchymal progenitor cells give rise to many cell lineages, but their molecular requirements for self-renewal and lineage decisions are incompletely understood. In this study, we show that their survival critically relies on the redundantly acting SoxC transcription factors Sox4, Sox11 and Sox12. The more SoxC alleles that are deleted in mouse embryos, the more severe and widespread organ hypoplasia is. SoxC triple-null embryos die at midgestation unturned and tiny, with normal patterning and lineage specification, but with massively dying neural and mesenchymal progenitor cells. Specific inactivation of SoxC genes in neural and mesenchymal cells leads to selective apoptosis of these cells, suggesting SoxC cell-autonomous roles. Tead2 functionally interacts with SoxC genes in embryonic development, and is a direct target of SoxC proteins. SoxC genes therefore ensure neural and mesenchymal progenitor cell survival, and function in part by activating this transcriptional mediator of the Hippo signalling pathway. Neural and mesenchymal progenitor cells arise in developing embryos from ectoderm, mesoderm and endoderm. As they actively self-renew, neural cells also give rise to all neuronal and glial cell types, whereas mesenchymal cells form stromal cells, osteoblasts, chondrocytes, adipocytes and myoblasts, among other cell types. These multipotent progenitor cells thereby have essential roles in organogenesis. They are still present in adult tissues, but are much less abundant than in embryonic tissues. They are then typically referred to as neural and mesenchymal stem cells. Evidence is increasing that they have key roles in normal tissue turnover and repair, and in the development of such diseases as cancers [1] , [2] , [3] . Active research is conducted worldwide to decipher the key features of these cells and their molecular regulation, not only to understand the basis of developmental, physiological and pathological processes but also because of the great promise that these cells could be used in therapies for many types of acquired and inherited diseases. However, many questions remain to be answered regarding the identity and regulation of these cells. Sox genes form a family of 20 in mammals [4] , [5] . They code for transcription factors featuring a high-mobility-group DNA-binding domain closely related to that of the male sex-determining protein Sry. Many have been shown to have master roles in the fate determination of specific cell types. For instance, Sox2 specifies the identity of embryonic stem cells in concert with Oct3/4, Klf4 and c-Myc [6] ; Sry and Sox9 specify Sertoli cell fate and differentiation [7] ; Sox5, Sox6 and Sox9 function together to specify the fate and differentiation of chondrocytes [8] ; and Sox18 specifies lymphatic endothelial cells [9] . The Sox family is divided into eight groups, A to H, according to protein identity. Sox4, Sox11 and Sox12 form the SoxC group [10] . They share a high degree of identity in the high-mobility-group domain, as well as in a group-specific transactivation domain [11] , [12] . Yet, sequence divergence within the latter domain explains that Sox11 is up to an order of magnitude more potent than Sox12 in activating reporter constructs in cultured cells, and that Sox4 exhibits an intermediate level of activity. Studies in mouse embryos have demonstrated that the three genes stand out by their high and concomitant expression in multipotent neural and mesenchymal progenitors [11] , [12] , [13] , [14] . As these cells differentiate, SoxC genes remain expressed only in a few cell lineages in a partially overlapping manner. Roles for SoxC genes in neural and mesenchymal progenitors are, however, yet to be demonstrated. Previous functional studies have revealed that Sox4 −/− mice die at embryonic day 14 (E14) from a heart outflow tract malformation referred to as common trunk, and from incomplete ventricular septation, but they seem normal otherwise [15] . Sox11 −/− mice die shortly after birth, with heart malformations similar to, but less severe than, those of Sox4 −/− mice [14] . They also exhibit internal organ malformations, including dysgenesis of the anterior eye segment, hypoplastic lungs and undermineralized bones and lack the spleen. Notably, the affected cell types have not been described in either mutant and the cellular and molecular mechanisms underlying these defects are unknown. Additional studies have shown that Sox4 is required to facilitate differentiation of T and B lymphocytes [15] , [16] , pancreatic β-cells [17] and osteoblasts [18] , but the mechanisms remain unclear. Defects in the central or peripheral nervous system were not described in Sox4 −/− and Sox11 −/− mice, but gene knockdown experiments in the chicken embryo have suggested that Sox4 and Sox11 function in redundancy to promote pan-neuronal marker gene expression [19] . However, no data were provided in this study on Sox4 and Sox11 single-gene knockdowns to support the conclusion of gene redundancy. Sox12 −/− mice are viable, fertile and do not exhibit any obvious defect [12] , leaving Sox12 as one of only two Sox genes with no known function in vivo . Recent studies have shown upregulation of Sox4 or Sox11 in various types of cancers, including medulloblastomas [20] , gliomas [21] , [22] , non-B-cell lymphomas [23] and prostate [24] and colon cancer [25] . These genes have been reported to be indicators of either good or poor prognosis in cancer patients, and to have possible but yet unclear roles in metastatic invasion, cell survival, apoptosis and differentiation [22] , [26] , [27] , [28] . This survey of literature reveals that the roles of SoxC genes are still poorly understood and likely to be context dependent. On the basis of their strong and overlapping expression in neural and mesenchymal progenitors, we hypothesized that SoxC genes have important functions in these cells that were not apparent in single knockout experiments because of gene redundancy. We tested this hypothesis by generating mouse embryos lacking increasing numbers of SoxC alleles in a global or cell-type-specific manner. We find that the three genes are redundantly required for successful organogenesis. They primarily control survival of neural and mesenchymal progenitors and function at least in part by activating the gene for Tead2, a transcriptional mediator of the Hippo pathway. SoxC genes fulfil key roles in organogenesis We tested the possibility that the three SoxC genes exert important redundant functions in vivo by generating mice harbouring all combinations of SoxC- null alleles. We used a previously described Sox4 conditional null allele [29] ( Sox4 fl ) in combination with a new Sox11 conditional null allele ( Sox11 fl ; Supplementary Fig. S1 ) and a new Sox12- null allele ( Sox12 − ; Supplementary Fig. S2 ). We recombined the conditional alleles in the germ line of male and female breeders using PrmCre [30] and Zp3Cre [31] transgenes, respectively, and thereby obtained embryos containing wild-type and/or SoxC- null alleles ( Supplementary Fig. S3 ). Sox4 +/− and Sox11 +/− mice were indistinguishable from wild-type littermates, as reported [14] , [15] . In contrast, Sox4 +/− 11 +/− mice died on birth, similar to Sox11 −/− littermates ( Fig. 1a , Supplementary Fig. S4 and Supplementary Table S1 ). Both types of mice displayed an incomplete septation of the heart ventricles. In addition, the aorta and pulmonary arteries were distinct in Sox4 +/− 11 +/− mice but both originated in the right ventricle. They were fused in Sox11 −/− mice and also originated in the right ventricle ( Fig. 1b , Supplementary Fig. S4 and Supplementary Table S1 ). These two types of outflow tract malformations are known as double-outlet right ventricle and common trunk, respectively, and reflect endocardial ridge dysgenesis with variable severity. Both mouse types also had similar skeletal malformations: hypoplastic sternebrae, unfused lumbar vertebral bodies and hypomineralized skull ( Fig. 1c,d and Supplementary Fig. S4 ). About 50% Sox11 −/− and Sox4 +/− 11 +/− mice had omphalocele. All Sox11 −/− mice were asplenic, and about 60% Sox4 +/− 11 +/− mice were hyposplenic. All Sox11 −/− newborns had microphthalmia and open eyelids and 40% had a cleft palate, cleft lips and a kinked tail, whereas no Sox4 +/− 11 +/− littermates had these defects ( Supplementary Table S1 ). Sox4 +/− 11 +/− mice thus exhibited a subset of the pleiotropic malformations of Sox11 −/− mice, and these malformations were generally milder. 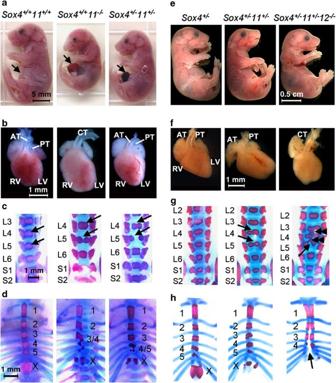Figure 1:SoxCgenes functionally interact with each other in multiple developmental processes. (a) E18.5Sox4+/−11+/−andSox11−/−littermates often display omphalocele (arrows), andSox11−/−mice have open eyelids and cleft lips. (b) E18.5Sox11−/−mice have a common arterial trunk (CT), andSox4+/−11+/−mice have the arterial (AT) and pulmonary (PT) trunks emerging from the right ventricle (RV). LV, left ventricle. (c) E18.5 fetus skeletal preparations, in which non-mineralized cartilage is stained with Alcian blue and mineralized bone and cartilage with Alizarin red, reveal that vertebral bodies (arrows, shown from the third lumbar vertebra—L3—to the second sacral vertebra—S2) are well formed in control mice, but that L4 and L5 are duplicated inSox11−/−andSox4+/−11+/−mice. (d) Skeletal preparations of the thoracic cage show that the five sternebrae (numbers 1–5) and the xyphoid process (X) are mineralized and distinct in control mice, whereas the last two or three sternebrae and the xyphoid process ofSox11−/−andSox4+/−11+/−mice are misshapen and irregularly mineralized. (e) E18.5Sox4+/−, Sox4+/−11+/−andSox4+/−11+/−12−/−littermates look normal. (f)Sox4+/−andSox4+/−11+/−fetuses have distinct aortic and pulmonary trunks, butSox4+/−11+/−12−/−littermates have a common trunk. (g) SeveralSox4+/−11+/−12−/−lumbar vertebral bodies are fused (double arrowheads) along the antero-posterior axis, in addition to being duplicated (arrows) along the midline. (h) Skeletal preparations show that the sternal bars ofSox4+/−11+/−12−/−embryos are barely fused at the midline (arrow) and that the xyphoid process (X) and fifth (5) sternebra are hardly, if at all, mineralized. Figure 1: SoxC genes functionally interact with each other in multiple developmental processes. ( a ) E18.5 Sox4 +/− 11 +/− and Sox11 −/− littermates often display omphalocele (arrows), and Sox11 −/− mice have open eyelids and cleft lips. ( b ) E18.5 Sox11 −/− mice have a common arterial trunk (CT), and Sox4 +/− 11 +/− mice have the arterial (AT) and pulmonary (PT) trunks emerging from the right ventricle (RV). LV, left ventricle. ( c ) E18.5 fetus skeletal preparations, in which non-mineralized cartilage is stained with Alcian blue and mineralized bone and cartilage with Alizarin red, reveal that vertebral bodies (arrows, shown from the third lumbar vertebra—L3—to the second sacral vertebra—S2) are well formed in control mice, but that L4 and L5 are duplicated in Sox11 −/− and Sox4 +/− 11 +/− mice. ( d ) Skeletal preparations of the thoracic cage show that the five sternebrae (numbers 1–5) and the xyphoid process (X) are mineralized and distinct in control mice, whereas the last two or three sternebrae and the xyphoid process of Sox11 −/− and Sox4 +/− 11 +/− mice are misshapen and irregularly mineralized. ( e ) E18.5 Sox4 +/− , Sox4 +/− 11 +/− and Sox4 +/− 11 +/− 12 −/− littermates look normal. ( f ) Sox4 +/− and Sox4 +/− 11 +/− fetuses have distinct aortic and pulmonary trunks, but Sox4 +/− 11 +/− 12 −/− littermates have a common trunk. ( g ) Several Sox4 +/− 11 +/− 12 −/− lumbar vertebral bodies are fused (double arrowheads) along the antero-posterior axis, in addition to being duplicated (arrows) along the midline. ( h ) Skeletal preparations show that the sternal bars of Sox4 +/− 11 +/− 12 −/− embryos are barely fused at the midline (arrow) and that the xyphoid process (X) and fifth (5) sternebra are hardly, if at all, mineralized. Full size image Sox12 −/− mice looked normal and were viable and fertile, as described [12] . Interestingly, however, inactivating Sox12 worsened the disease phenotype of Sox4 +/− 11 +/− mice. Many Sox4 +/− 11 +/− 12 −/− mice had an arterial common trunk, and all had aggravated sternal and vertebral malformations, compared with Sox4 +/− 11 +/− littermates ( Fig. 1e–h Supplementary Fig. S5 and Supplementary Table S1 ). Sox4 +/− 11 −/− mice died in utero between E14.5 and E16.5, with an arterial common trunk and hypoplastic myocardium and semilunar valves ( Supplementary Fig. S6 ). They had many other underdeveloped organs as well, such as eyes, lungs and skeleton, and were thus more severely affected than Sox4 +/− 11 +/− and Sox11 −/− mice. Sox4 +/− 11 −/− and Sox4 −/− 11 −/− embryos died around E10.5. At E9.5, Sox4 −/− 11 −/− embryos were similar, but more affected than Sox4 +/− 11 −/− littermates. They were tiny and unturned ( Fig. 2a–c ). The heart primordia had not fused. The neural tube was thin, undulated and rostrally open. Limbs were failing to bud, and somites were rudimentary. These embryos thus arrested their development around E8.5. Sox4 −/− 11 −/− 12 −/− littermates were slightly more affected ( Fig. 2d ). 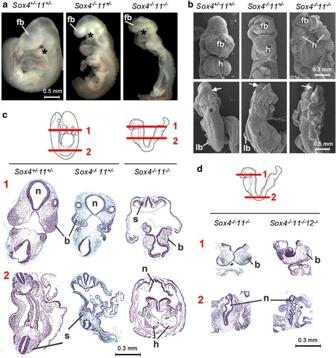Figure 2:SoxCgenes are necessary in early organogenesis. (a) Side views of E9.5Sox4−/−11+/−,Sox4−/−11+/−andSox4−/−11−/−littermates show that the latter two types of mutants are smaller and not fully turned. fb, forebrain; asterisk (*), branchial arches. (b) Scanning electron microscopy of E9.5 embryos. The top row shows ventral views of the head and heart, and the bottom row shows dorsal views. Note the lack of heart (h) coiling in theSox4−/−11+/−embryo, cardia bifida in theSox4−/−11−/−embryo and incomplete closure of the neural tube in the cephalic region (arrows) inSox4−/−11+/−andSox4−/−11−/−embryos. lb, limb bud. (c) Histology sections of E9.5 embryos made as indicated by the schematics and stained with haematoxylin and eosin show that theSox4−/−11+/−andSox4−/−11−/−branchial arch mesenchyme (b) is loose and small. TheSox4−/−11−/−neural tube (n) is thin and wavy. Somites (s) are small. Heart primordia (h) are not fused.Sox4−/−11+/−embryos are partially turned, andSox4−/−11−/−embryos are not turned. (d) Histology sections show that the neural tube (n) is thinner and wavier in E9.5Sox4−/−11−/−12−/−embryos than inSox4−/−11−/−littermates, whereas the first branchial arch (b) mesenchyme is similar in size and degree of cellularity in the two types of embryos. Figure 2: SoxC genes are necessary in early organogenesis. ( a ) Side views of E9.5 Sox4 −/− 11 +/− , Sox4 −/− 11 +/− and Sox4 −/− 11 −/− littermates show that the latter two types of mutants are smaller and not fully turned. fb, forebrain; asterisk (*), branchial arches. ( b ) Scanning electron microscopy of E9.5 embryos. The top row shows ventral views of the head and heart, and the bottom row shows dorsal views. Note the lack of heart (h) coiling in the Sox4 −/− 11 +/− embryo, cardia bifida in the Sox4 −/− 11 −/− embryo and incomplete closure of the neural tube in the cephalic region (arrows) in Sox4 −/− 11 +/− and Sox4 −/− 11 −/− embryos. lb, limb bud. ( c ) Histology sections of E9.5 embryos made as indicated by the schematics and stained with haematoxylin and eosin show that the Sox4 −/− 11 +/− and Sox4 −/− 11 −/− branchial arch mesenchyme (b) is loose and small. The Sox4 −/− 11 −/− neural tube (n) is thin and wavy. Somites (s) are small. Heart primordia (h) are not fused. Sox4 −/− 11 +/− embryos are partially turned, and Sox4 −/− 11 −/− embryos are not turned. ( d ) Histology sections show that the neural tube (n) is thinner and wavier in E9.5 Sox4 −/− 11 −/− 12 −/− embryos than in Sox4 −/− 11 −/− littermates, whereas the first branchial arch (b) mesenchyme is similar in size and degree of cellularity in the two types of embryos. Full size image The fact that phenotypic severity increased in parallel with the number of SoxC- deleted alleles demonstrates that the three genes functionally interact with each other to fulfil key roles in organogenesis. SoxC genes control neural and mesenchymal cell survival To identify the original nature of the defects of Sox4 −/− 11 −/− 12 −/− embryos, we first examined the expression pattern of SoxC genes in wild-type embryos when these mutants start failing ( Supplementary Fig. S7 ). We found all three genes expressed throughout most embryonic structures, indicating that these genes could directly control most organogenetic processes. We then analysed the expression of genes involved in cell lineage determination and embryo patterning in Sox4 −/− 11 −/− embryos. We found that neural tube markers were properly expressed along the dorsoventral ( Pax7 , Ptc1 , Shh ) and anteroposterior axes ( Otx2 , Fgf8 , HoxB9 ) ( Fig. 3a,b ). Similarly, notochord ( Shh , Brachyury ), sclerotome ( Pax1 ), lateral/ventral mesoderm ( Bmp4 ), myotome ( Myf5 ) and dermomyotome ( Pax7 ) markers and regulatory genes were also normally expressed ( Fig. 3a ). 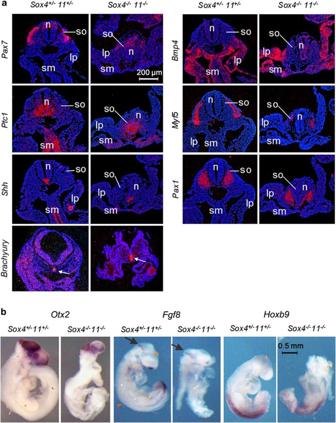Figure 3: Embryo axial patterning and tissue specification are not affected bySoxCinactivation. (a) RNAin situhybridizations of E9.5 embryo sections demonstrate thatPax7(dorsal neural tube and dermomyotome),Ptc1(ventral neural tube, paraxial mesoderm, splanchnic mesoderm),Shh(notochord and neural floor plate),Brachyury(notochord),Bmp4(lateral/ventral mesoderm),Myf5(myotome) andPax1(sclerotome) are expressed normally inSox4−/−11−/−embryos. lp, lateral plate mesoderm; n, neural tube; so, somite, sm, splanchnic mesoderm. RNA signals are seen in red and cell nuclei are stained in blue with the Hoechst dye 33258. (b) Whole-mount RNAin situhybridizations show that the expression domains ofOtx2(forebrain),Fgf8(midbrain, arrows) andHoxb9(spinal cord) are maintained in E9.5Sox4−/−11−/−embryos. Figure 3: Embryo axial patterning and tissue specification are not affected by SoxC inactivation. ( a ) RNA in situ hybridizations of E9.5 embryo sections demonstrate that Pax7 (dorsal neural tube and dermomyotome), Ptc1 (ventral neural tube, paraxial mesoderm, splanchnic mesoderm), Shh (notochord and neural floor plate), Brachyury (notochord), Bmp4 (lateral/ventral mesoderm), Myf5 (myotome) and Pax1 (sclerotome) are expressed normally in Sox4 −/− 11 −/− embryos. lp, lateral plate mesoderm; n, neural tube; so, somite, sm, splanchnic mesoderm. RNA signals are seen in red and cell nuclei are stained in blue with the Hoechst dye 33258. ( b ) Whole-mount RNA in situ hybridizations show that the expression domains of Otx2 (forebrain), Fgf8 (midbrain, arrows) and Hoxb9 (spinal cord) are maintained in E9.5 Sox4 −/− 11 −/− embryos. Full size image We next analysed cell death and proliferation. TdT-mediated dUTP nick end labeling assays revealed a drastic increase in cell death in the neural tube, branchial arches and somites of E9.5 Sox4 −/− 11 −/− embryos ( Fig. 4a ). To rule out that cell death was a consequence of global embryo failure, we specifically inactivated Sox4 and Sox11 in specific cell types ( Fig. 4b–e ). Neuronal-specific inactivation using a Brn4Cre [32] transgene resulted in a strong and selective increase in cell death in the neural tube ( Fig. 4b ). Similarly, specific inactivation in the neural crest using a Wnt1Cre [33] transgene did not prevent cell delamination from the neural tube and migration into specific sites in the embryos, as proven by cell tracking with the Rosa26 lacZ Cre reporter [34] , but led to massive cell death in branchial arches ( Fig. 4c ). Specific inactivation in limb bud mesenchyme using a Prx1Cre transgene [35] resulted in a large increase in cell death in this tissue ( Fig. 4d ). Furthermore, inactivation in primary limb bud cells using Cre adenoviral infection also resulted in increased cell death ( Fig. 4f ). 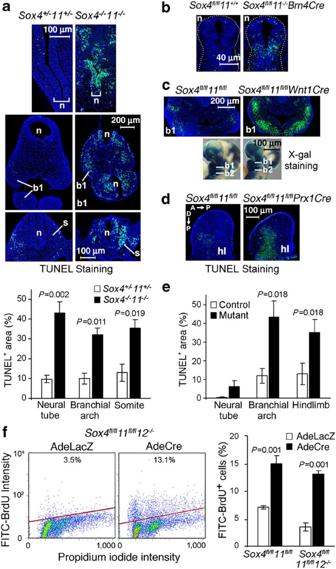Figure 4:SoxCgenes are required for neural and mesenchymal cell survival. (a) TdT-mediated dUTP nick end labeling (TUNEL) assay in E9.5 embryo sections shows increased cell death in the neural tube (n), first branchial arch mesenchyme (b1) and somites (s) ofSox4−/−11−/−embryos compared withSox4+/−11+/−littermates. Cell nuclei are rendered blue with 4,6-diamidino-2-phenylindole (DAPI), and apoptotic bodies fluoresce in green. The percentage of TUNEL versus DAPI signal in areas of interest is shown as average with standard deviation obtained for three sections in each of three embryos per genotype. Statistical significance was determined using a Student's two-tailed, pairedt-test. (b) TUNEL assay in embryo sections shows increased cell death in the neural tube (n) of E10.5Sox4fl/fl11−/−Brn4Creembryos. (c) TUNEL assay in embryo sections shows increased cell death in the branchial arch mesenchyme (b1) of E10.5Sox4fl/fl11fl/flWnt1Creembryos. 5-bromo-4-chloro-3-indolyl-β-D-galactoside staining ofSox4fl/fl11fl/flandSox4fl/fl11fl/flR26lacZWnt1Crelittermates shows that neural crest cells have migrated to proper sites in the first (b1) and second (b2) branchial arches of the mutants. (d) TUNEL assay in embryo sections shows increased cell death in the hindlimb mesenchyme (hl) of E11.5Sox4fl/fl11fl/flPrx1Creembryos. The antero-posterior (A→P) and proximo–distal (P→D) axes of limb buds are indicated. (e) Percentage of TUNEL-positive cells or area in control and mutant tissues of interest. Quantification was carried out as described in panel a. (f) Flow cytometry TUNEL assay shows more dead cells inSox4fl/fl11fl/flandSox4fl/fl11fl/fl12−/−primary limb bud cell cultures treated with Cre-expressing adenovirus (AdeCre) than in AdeLacZ-treated control cultures. Left panels, fluorescence-activated cell sorting profiles of representative samples. The percentage of dead cells (BrdU+, above the red line) is indicated. Right panel, average with standard deviation of data obtained from three independent experiments. Statistical significance was determined using a Student's two-tailed, pairedt-test. Figure 4: SoxC genes are required for neural and mesenchymal cell survival. ( a ) TdT-mediated dUTP nick end labeling (TUNEL) assay in E9.5 embryo sections shows increased cell death in the neural tube (n), first branchial arch mesenchyme (b1) and somites (s) of Sox4 −/− 11 −/− embryos compared with Sox4 +/− 11 +/− littermates. Cell nuclei are rendered blue with 4,6-diamidino-2-phenylindole (DAPI), and apoptotic bodies fluoresce in green. The percentage of TUNEL versus DAPI signal in areas of interest is shown as average with standard deviation obtained for three sections in each of three embryos per genotype. Statistical significance was determined using a Student's two-tailed, paired t- test. ( b ) TUNEL assay in embryo sections shows increased cell death in the neural tube (n) of E10.5 Sox4 fl/fl 11 −/− Brn4Cre embryos. ( c ) TUNEL assay in embryo sections shows increased cell death in the branchial arch mesenchyme (b1) of E10.5 Sox4 fl/fl 11 fl/fl Wnt1Cre embryos. 5-bromo-4-chloro-3-indolyl-β- D -galactoside staining of Sox4 fl/fl 11 fl/fl and Sox4 fl/fl 11 fl/fl R26 lacZ Wnt1Cre littermates shows that neural crest cells have migrated to proper sites in the first (b1) and second (b2) branchial arches of the mutants. ( d ) TUNEL assay in embryo sections shows increased cell death in the hindlimb mesenchyme (hl) of E11.5 Sox4 fl/fl 11 fl/fl Prx1Cre embryos. The antero-posterior (A→P) and proximo–distal (P→D) axes of limb buds are indicated. ( e ) Percentage of TUNEL-positive cells or area in control and mutant tissues of interest. Quantification was carried out as described in panel a. ( f ) Flow cytometry TUNEL assay shows more dead cells in Sox4 fl/fl 11 fl/fl and Sox4 fl/fl 11 fl/fl 12 −/− primary limb bud cell cultures treated with Cre-expressing adenovirus (AdeCre) than in AdeLacZ-treated control cultures. Left panels, fluorescence-activated cell sorting profiles of representative samples. The percentage of dead cells (BrdU + , above the red line) is indicated. Right panel, average with standard deviation of data obtained from three independent experiments. Statistical significance was determined using a Student's two-tailed, paired t -test. Full size image Phospho-histone-3 immunostaining and 5-bromodeoxyuridine (BrdU) incorporation assays showed a significant reduction in cell proliferation in the neural tube, branchial arches and somites of Sox4 −/− 11 −/− embryos ( Fig. 5a ). In contrast, specific inactivation of Sox4 and Sox11 in these structures in vivo or in corresponding primary cells in vitro did not alter cell proliferation ( Fig. 5b–e ). 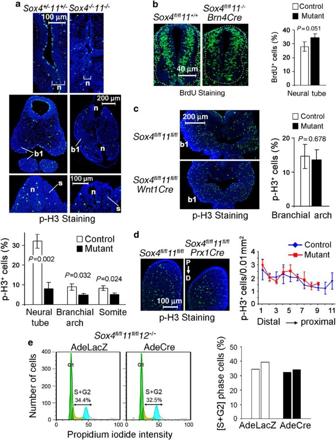Figure 5: The rate of cell proliferation is reduced inSox4−/−11−/−embryos, not in conditional mutants. (a) E9.5 embryo sections immunostained for phospho-histone-3 (p-H3, green signal) and counterstained with 4,6-diamidino-2-phenylindole (blue signal) show a lower rate of cell proliferation in the subventricular layer of the neural tube (n), first branchial arch (b1) and somitic mesenchyme (s) ofSox4−/−11−/−embryos than inSox4+/−11+/−littermates. The percentage of p-H3-positive cells is shown as the average with standard deviation for three sections in each of three embryos per genotype. Statistical significance was determined using a Student's two-tailed, pairedttest. (b) Immunostaining of BrdU incorporation (green signal) in E10.5Sox4fl/fl11+/+andSox4fl/fl11−/−Brn4Crelittermates. Quantification was carried out as described ina. (c) p-H3 staining of sections from E10.5Sox4fl/fl11fl/flandSox4fl/fl11fl/flR26lacZWnt1Crelittermates at the level of the first branchial arches (b1). Quantification was carried out as described ina. (d) p-H3 staining of hindlimb bud sections from E11.5Sox4fl/fl11fl/flandSox4fl/fl11fl/flPrx1Crelittermates. The number of p-H3-positive cells was calculated per 0.01 mm2in up to 11 consecutive layers drawn along the proximo–distal axis (P→D). The plot shows the averages with standard deviation of p-H3-positive cells per surface area in three adjacent sections for a representative experiment. (e) Analysis of cell-cycle distribution by propidium iodide staining of primary limb bud cells from E11.5Sox4fl/fl11fl/fl12−/−embryos 24 h after infection with AdeLacZ or AdeCre. Representative fluorescence-activated cell sorting profiles are shown. The percentages of cells in S and G2 phase are shown for two independent experiments. Figure 5: The rate of cell proliferation is reduced in Sox4 −/− 11 −/− embryos, not in conditional mutants. ( a ) E9.5 embryo sections immunostained for phospho-histone-3 (p-H3, green signal) and counterstained with 4,6-diamidino-2-phenylindole (blue signal) show a lower rate of cell proliferation in the subventricular layer of the neural tube (n), first branchial arch (b1) and somitic mesenchyme (s) of Sox4 −/− 11 −/− embryos than in Sox4 +/− 11 +/− littermates. The percentage of p-H3-positive cells is shown as the average with standard deviation for three sections in each of three embryos per genotype. Statistical significance was determined using a Student's two-tailed, paired t test. ( b ) Immunostaining of BrdU incorporation (green signal) in E10.5 Sox4 fl/fl 11 +/+ and Sox4 fl/fl 11 −/− Brn4Cre littermates. Quantification was carried out as described in a . ( c ) p-H3 staining of sections from E10.5 Sox4 fl/fl 11 fl/fl and Sox4 fl/fl 11 fl/fl R26 lacZ Wnt1Cre littermates at the level of the first branchial arches (b1). Quantification was carried out as described in a . ( d ) p-H3 staining of hindlimb bud sections from E11.5 Sox4 fl/fl 11 fl/fl and Sox4 fl/fl 11 fl/fl Prx1Cre littermates. The number of p-H3-positive cells was calculated per 0.01 mm 2 in up to 11 consecutive layers drawn along the proximo–distal axis (P→D). The plot shows the averages with standard deviation of p-H3-positive cells per surface area in three adjacent sections for a representative experiment. ( e ) Analysis of cell-cycle distribution by propidium iodide staining of primary limb bud cells from E11.5 Sox4 fl/fl 11 fl/fl 12 −/− embryos 24 h after infection with AdeLacZ or AdeCre. Representative fluorescence-activated cell sorting profiles are shown. The percentages of cells in S and G2 phase are shown for two independent experiments. Full size image We conclude that SoxC genes are not needed for embryo patterning and cell lineage specification, but are required for cell survival in such tissues as neural tube, branchial arch, somite and limb bud. Effects on cell proliferation are likely to be secondary. At the time of analysis, most cells in these tissues are at the neural and mesenchymal progenitor stages. Their high-level expression of SoxC genes strongly suggests that the genes function in a cell-autonomous manner. Furthermore, widespread death of progenitors likely caused the catastrophic failure of SoxC mutant embryos. SoxC genes function upstream of Tead2 To identify how SoxC genes mediate their functions, we screened RNA isolated from Sox4 fl/fl 11 fl/fl primary limb bud cells treated with Cre- or LacZ- expressing adenovirus in gene expression microarrays. As SoxC proteins are transcriptional activators, we focused on genes downregulated in SoxC mutant cells. Expression of 38 genes was downregulated at least twofold ( Supplementary Table S2 ). Tead2 figured in the top 10 and we chose to focus on this gene because it is the only one known to promote cell survival during organogenesis. Tead2 and its family members encode transcription factors that associate with YAP and TAZ coactivators to mediate cell survival and proliferation downstream of the Hippo signalling pathway [36] . This pathway intrinsically controls organ size in development and tumour growth. Tead2 -null mice occasionally show a neural tube closure defect [37] , but are otherwise normal. Inactivation of Tead2 , however, aggravates the phenotype of Tead1 -null mice and results in an embryo phenotype strikingly similar to that of SoxC -null embryos [38] . We confirmed that expression of Tead2 , but not expression of its family members, was significantly downregulated in SoxC mutant embryos, primary limb bud cells and undifferentiated osteoblasts, using real-time reverse transcription–PCR and RNA hybridization in situ ( Fig. 6a–c and Supplementary Fig. S8a–d ). We then determined whether Tead2 downregulation could contribute to the phenotype of SoxC mutants. We found that Tead2 −/− Sox4 +/− 11 +/− embryos had a significantly higher incidence of heart double-outlet right ventricle and ventricular septation defects than Tead2 −/− and Sox4 +/− 11 +/− littermates and also had more severe and more frequent vertebral malformations ( Fig. 6d,e ). A gradual increase in the incidence of mesenchymal cell death was measured around the notochord of E11.5 embryos, as progressively more Tead2 and SoxC alleles were deleted ( Fig. 6f ). This rise in cell death was specific to the lumbar region, and thus likely explains the increased severity and occurrence of lumbar vertebral malformations seen in Tead2/SoxC compound mutants. We next tested whether forced expression of Tead2 would be sufficient to rescue the cell death phenotype caused by SoxC inactivation. We found that exogenous expression of wild-type Tead2 in undifferentiated primary osteoblasts was insufficient to prevent cell death on SoxC inactivation, but that a constitutively active form of Tead2, obtained by fusing Tead2 with the YAP transactivation domain [39] , was able to fully rescue this phenotype ( Fig. 6g ). Together, these data thus strongly suggest that SoxC genes control cell survival upstream of Tead2 and the Hippo pathway. 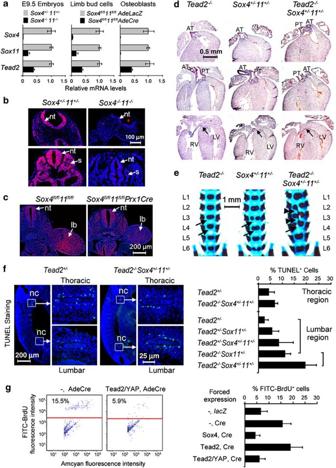Figure 6:Tead2is expressed and functions downstream of theSoxCgenes. (a) Quantitative real-time reverse transcription–PCR shows RNA levels ofSox4,Sox11andTead2relative toGapdhin control and mutant samples. Data are presented as average with standard deviation from three independent samples. Control and mutant data are statistically different (P<0.002, two-tailed Student'st-test). (b) RNAin situhybridization of E9.5 embryo sections showsTead2downregulation inSox4−/−11−/−neural tissue (nt) and somites (s). (c) RNAin situhybridization showsTead2downregulation in limb bud mesenchyme (lb) of E10.5Sox4fl/fl11fl/flPrx1Cremutants, but not in neural tube (nt) and other sites. (d) Frontal sections show a normal heart in E18.5Tead2−/−fetuses. OneSox4+/−11+/−embryo (out of 4:n=4) and twoSox4+/−11+/−Tead2+/−embryos (n=9) had ventricular septation defect. AllTead2−/−Sox4+/−11+/−littermates (n=7) had this defect (arrow) and arterial (AT) and pulmonary (PT) trunks arising from the right ventricle. The septation defect is more frequent inSox4+/−11+/−Tead2−/−than inSox4+/−11+/−andSox4+/−11+/−Tead2+/−fetuses (P=0.024 and 0.003, respectively, two-tailed, Fisher's exact test). (e) Skeletal preparations show that allTead2−/−fetuses (n=8) had normal vertebral bodies (arrows). AllSox4+/−11+/−(n=4),Sox4+/−11+/−Tead2+/−(n=9) andSox4+/−11+/−Tead2−/−littermates (n=7) had duplication of several lumbar vertebral bodies, and sixSox4+/−11+/−Tead2−/−fetuses also had vertebral body antero-posterior fusions (double arrowheads). The latter phenotype was significantly different from that of littermates (P≤0.015, two-tailed, Fisher's exact test). (f) TdT-mediated dUTP nick end labeling assay in E11.5 embryo sections shows increased cell death around the notochord in the lumbar, but not in the thoracic region, inSox4+/−11+/−Tead2−/−embryos compared with control littermates. Left, representative pictures. Right, average with standard deviation of data from three embryos per genotype. Brackets link statistically different data (P-value <0.01, Student's two-tailed, pairedt-test). (g) Apoptosis assay inSox4fl/fl11fl/flandSox4fl/fl11fl/fl12−/−osteoblasts. Cells were treated withAdeLacZorAdeCreafter transfection with expression plasmids for Amcyan protein and no protein (−), Sox4, Tead2 or Tead2/YAP. Left, representative fluorescence-activated cell sorting profiles. The percentage of Amcyan+dying cells is indicated. Right, average with standard deviation of data from three independent experiments. Sox4,Cre and Tead2/YAP,Cre data are statistically different from [−,Cre] data (P<0.01, two-tailed Student'st-test). Figure 6: Tead2 is expressed and functions downstream of the SoxC genes. ( a ) Quantitative real-time reverse transcription–PCR shows RNA levels of Sox4 , Sox11 and Tead2 relative to Gapdh in control and mutant samples. Data are presented as average with standard deviation from three independent samples. Control and mutant data are statistically different ( P <0.002, two-tailed Student's t -test). ( b ) RNA in situ hybridization of E9.5 embryo sections shows Tead2 downregulation in Sox4 −/− 11 −/− neural tissue (nt) and somites (s). ( c ) RNA in situ hybridization shows Tead2 downregulation in limb bud mesenchyme (lb) of E10.5 Sox4 fl/fl 11 fl/fl Prx1Cre mutants, but not in neural tube (nt) and other sites. ( d ) Frontal sections show a normal heart in E18.5 Tead2 −/− fetuses. One Sox4 +/− 11 +/− embryo (out of 4: n =4) and two Sox4 +/− 11 +/− Tead2 +/− embryos ( n =9) had ventricular septation defect. All Tead2 −/− Sox4 +/− 11 +/− littermates ( n =7) had this defect (arrow) and arterial (AT) and pulmonary (PT) trunks arising from the right ventricle. The septation defect is more frequent in Sox4 +/− 11 +/− Tead2 −/− than in Sox4 +/− 11 +/− and Sox4 +/− 11 +/− Tead2 +/− fetuses ( P =0.024 and 0.003, respectively, two-tailed, Fisher's exact test). ( e ) Skeletal preparations show that all Tead2 −/− fetuses ( n =8) had normal vertebral bodies (arrows). All Sox4 +/− 11 +/− ( n =4), Sox4 +/− 11 +/− Tead2 +/− ( n =9) and Sox4 +/− 11 +/− Tead2 −/− littermates ( n =7) had duplication of several lumbar vertebral bodies, and six Sox4 +/− 11 +/− Tead2 −/− fetuses also had vertebral body antero-posterior fusions (double arrowheads). The latter phenotype was significantly different from that of littermates ( P ≤0.015, two-tailed, Fisher's exact test). ( f ) TdT-mediated dUTP nick end labeling assay in E11.5 embryo sections shows increased cell death around the notochord in the lumbar, but not in the thoracic region, in Sox4 +/− 11 +/− Tead2 −/− embryos compared with control littermates. Left, representative pictures. Right, average with standard deviation of data from three embryos per genotype. Brackets link statistically different data ( P -value <0.01, Student's two-tailed, paired t -test). ( g ) Apoptosis assay in Sox4 fl/fl 11 fl/fl and Sox4 fl/fl 11 fl/fl 12 −/− osteoblasts. Cells were treated with AdeLacZ or AdeCre after transfection with expression plasmids for Amcyan protein and no protein (−), Sox4, Tead2 or Tead2/YAP. Left, representative fluorescence-activated cell sorting profiles. The percentage of Amcyan + dying cells is indicated. Right, average with standard deviation of data from three independent experiments. Sox4,Cre and Tead2/YAP,Cre data are statistically different from [−,Cre] data ( P <0.01, two-tailed Student's t -test). Full size image Tead2 is a direct target of SoxC proteins To test whether Tead2 is a direct target of SoxC proteins, we first searched for putative regulatory regions in the form of highly conserved, non-coding, non-repetitive sequences within and around Tead2 ( Fig. 7a ). The only regions fitting these criteria were a 105 bp sequence encompassing the promoter and first exon (referred to as PE1), and a 500 bp sequence in the middle of the first intron (InS). We constructed reporter genes and found that each SoxC protein robustly activated reporters containing both InS and PE1 sequences in transiently transfected Cos1 cells ( Fig. 7b,c ). Sequence analysis revealed two putative Sox-binding sites in PE1, and three in InS ( Fig. 7a,d ). Sox4 efficiently bound to all but one of these sites in an electrophoretic mobility shift assay ( Fig. 7e ). Mutations that specifically abolished Sox4 binding in electrophoretic mobility shift assay also reduced reporter transactivation, strongly suggesting that SoxC proteins directly activate these reporters ( Fig. 7c ). To test whether these factors directly transactivate Tead2 in vivo , we performed a chromatin immunoprecipitation assay in C3H-10T1/2 mesenchymal cells expressing FLAG-Sox proteins. A FLAG antibody specifically precipitated PE1- and InS-containing chromatin fragments in FLAG-SoxC-expressing cells. Interestingly, an RNA polymerase II antibody specifically precipitated PE1-containing chromatin fragments only from FLAG-SoxC-expressing cells ( Fig. 7f ). These data thus demonstrate that Tead2 is a direct target of SoxC proteins. 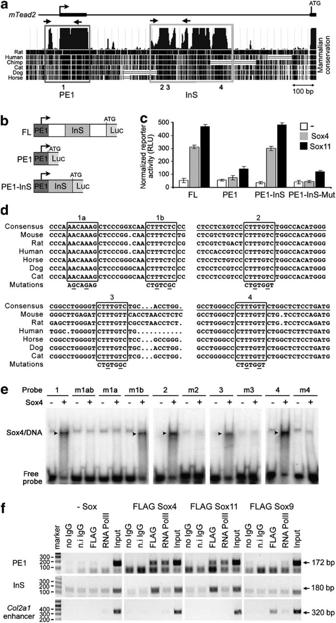Figure 7: SoxC proteins directly activateTead2. (a) Schematic of the mouseTead2locus from upstream of the transcription start site (angled arrow) to downstream of the translation start site (ATG) in the second exon, and analysis of mammalian conservation. Highly conserved, non-coding sequences were found in the promoter and first exon (PE1 box) and in the first intron (InS box). No other highly conserved region was found in otherTead2introns or in the agenic region aroundTead2(data not shown). Arrows, position of primers used in chromatin immunoprecipitation assay. Numbers 1–4 indicate the position of Sox-binding sites. (b)Tead2reporters were made by cloning the indicatedTead2sequences upstream of the firefly luciferase gene. (c) Transient transfection of Cos-1 cells withTead2reporters and expression vectors for Sox4, Sox11 or no protein (−). Reporter activities (RLU, relative luciferase units) were normalized for transfection efficiency and are presented as the average with standard deviation of data obtained from three independent cultures. Constructs bearing PE1+InS are significantly activated by SoxC proteins (P<0.001, Student'st-test), unless the SoxC-binding sites are mutated (PE1+InS-Mut). (d) ClustalW alignment of sequences encompassing putative SoxC-binding sites in several mammalian genomes. These sites are boxed. These sequences and mutant versions, as indicated, were used to generate electrophoretic mobility shift assay probes. (e) Electrophoretic mobility shift assay withTead2probes and protein extracts from Cos-1 cells transfected with a Sox4 expression plasmid. Sox4 binds to all wild-type probes (arrowhead), but not to mutant probes, except m1b. (f) Chromatin immunoprecipitation assay of SoxC proteins binding to endogenousTead2. Chromatin extracts from C3H-10T1/2 cells transiently expressing FLAG-Sox proteins were precipitated in the absence (no IgG) or presence of non-immune (n.i.) rabbit IgG, RNA polymerase II antibody or FLAG antibody. PCR products from immunoprecipitated chromatin and input are shown on resolution by agarose gel electrophoresis. DNA markers and the size of PCR products are shown. Figure 7: SoxC proteins directly activate Tead2 . ( a ) Schematic of the mouse Tead2 locus from upstream of the transcription start site (angled arrow) to downstream of the translation start site (ATG) in the second exon, and analysis of mammalian conservation. Highly conserved, non-coding sequences were found in the promoter and first exon (PE1 box) and in the first intron (InS box). No other highly conserved region was found in other Tead2 introns or in the agenic region around Tead2 (data not shown). Arrows, position of primers used in chromatin immunoprecipitation assay. Numbers 1–4 indicate the position of Sox-binding sites. ( b ) Tead2 reporters were made by cloning the indicated Tead2 sequences upstream of the firefly luciferase gene. ( c ) Transient transfection of Cos-1 cells with Tead2 reporters and expression vectors for Sox4, Sox11 or no protein (−). Reporter activities (RLU, relative luciferase units) were normalized for transfection efficiency and are presented as the average with standard deviation of data obtained from three independent cultures. Constructs bearing PE1+InS are significantly activated by SoxC proteins ( P <0.001, Student's t -test), unless the SoxC-binding sites are mutated (PE1+InS-Mut). ( d ) ClustalW alignment of sequences encompassing putative SoxC-binding sites in several mammalian genomes. These sites are boxed. These sequences and mutant versions, as indicated, were used to generate electrophoretic mobility shift assay probes. ( e ) Electrophoretic mobility shift assay with Tead2 probes and protein extracts from Cos-1 cells transfected with a Sox4 expression plasmid. Sox4 binds to all wild-type probes (arrowhead), but not to mutant probes, except m1b. ( f ) Chromatin immunoprecipitation assay of SoxC proteins binding to endogenous Tead2 . Chromatin extracts from C3H-10T1/2 cells transiently expressing FLAG-Sox proteins were precipitated in the absence (no IgG) or presence of non-immune (n.i.) rabbit IgG, RNA polymerase II antibody or FLAG antibody. PCR products from immunoprecipitated chromatin and input are shown on resolution by agarose gel electrophoresis. DNA markers and the size of PCR products are shown. Full size image This study revealed that the three SoxC genes largely work in redundancy to fulfil essential functions from the onset of mouse organogenesis. They have a primary role in ensuring survival of early neural and mesenchymal cells, the progenitors of many cell lineages, and they function at least in part by directly targeting the gene for Tead2, a transcription factor involved in mediating the intrinsic organ growth function of the Hippo signalling pathway ( Fig. 8 ). 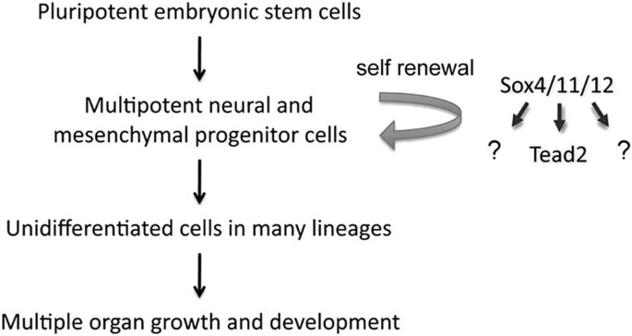Figure 8: Model for the roles ofSoxCgenes in organogenesis. Organogenesis starts as pluripotent embryonic stem cells develop into multipotent neural and mesenchymal cells. These progenitor cells are important for embryo growth and organogenesis through their ability to self-renew and give rise to many different cell types. This study demonstrated that SoxC proteins—Sox4, Sox11 and Sox12—have a primary role in ensuring the survival of these cells. They directly activate the gene for Tead2, a transcriptional mediator of the Hippo signalling pathway that is capable of mediating at least some of their cell survival functions. It is likely, however, that they also fulfil some of their functions through the activation of other genes that remain to be uncovered. Figure 8: Model for the roles of SoxC genes in organogenesis. Organogenesis starts as pluripotent embryonic stem cells develop into multipotent neural and mesenchymal cells. These progenitor cells are important for embryo growth and organogenesis through their ability to self-renew and give rise to many different cell types. This study demonstrated that SoxC proteins—Sox4, Sox11 and Sox12—have a primary role in ensuring the survival of these cells. They directly activate the gene for Tead2, a transcriptional mediator of the Hippo signalling pathway that is capable of mediating at least some of their cell survival functions. It is likely, however, that they also fulfil some of their functions through the activation of other genes that remain to be uncovered. Full size image Previous studies showed that Sox4 −/− mice die at E14 from heart malformations [15] . Sox11 −/− mice on the other hand die at birth with many hypoplastic or malformed organs [14] , whereas Sox12 −/− mice are viable and look normal [12] . Sox4 and Sox11 were reported to function in redundancy to promote differentiation of neuronal cells in the chicken embryo, but no data were provided to demonstrate this redundancy [19] . This study is thus the first to demonstrate that Sox12 has functions in vivo and that the three SoxC genes function redundantly in a multitude of developmental processes. On comparing mice with all combinations of SoxC- null alleles, we deduced that the dosage of SoxC alleles is critical for many of their functions and that each gene contributes to this dosage with a different weight. Inactivation of Sox12 slightly aggravates the phenotype of Sox4 +/− 11 +/− and Sox4 −/− 11 −/− embryos, but has otherwise no consequence, indicating that Sox12 provides minor contribution. We have not formally ruled out that the Sox12 protein may be present at a low level compared with Sox4 and Sox11 in wild-type mice. However, our previous observations [11] , [12] that the levels of the three SoxC RNAs are similar in most expression sites and that the Sox12 protein is a weak transactivator in vitro support the proposition that the minor contribution of Sox12 in vivo is due to the low transcriptional competence of its protein product. The aggravation of the phenotype of Sox4 +/− 11 +/− mutants on inactivation of Sox12 also rules out that Sox12 quenches the activity of its relatives by competing with them for target gene binding without providing comparable transactivation. We showed that Sox4 +/− 11 +/− mice are born with a subset of the defects of Sox11 −/− mice and that these defects are often milder than those of Sox11 −/− mice. In contrast, Sox4 −/− 11 +/− embryos are more affected than Sox4 +/− 11 −/− embryos in early organogenesis and are almost as severely affected as Sox4 −/− 11 −/− embryos. Thus, Sox4 has more weight in early functions and Sox11 in later functions. The differences between the two genes could be due to differences in expression levels or to differences in protein activities according to molecular contexts. We found that SoxC -null embryos are normal until E8.5, which demonstrates that SoxC genes are dispensable for embryo development through gastrulation. These embryos thus differ from Sox2 -null embryos, which die around E3.5, because Sox2 is required to maintain the pluripotent cells of the epiblast and extraembryonic ectoderm that later give rise to all embryonic and trophoblast cell types, respectively [40] . Epiblast pluripotent cells are used to derive embryonic stem cells in culture, and the latter have been shown to express Sox4 and Sox11 [41] . Interestingly, Sox4 was shown to directly control Sox2 expression downstream of transforming growth factor-β signalling in glioma-initiating stem cells in vitro [42] . However, we did not find a change in Sox2 expression in primary limb bud cell microarray experiments. In addition, SoxC -null embryos would die as early as Sox2 -null embryos, should the SoxC proteins critically control Sox2 expression in early embryos. SoxC proteins might thus control Sox2 expression in specific contexts, but not in the early embryo. We showed that SoxC -null embryos arrest in development at E8.5. This is when wild-type mouse embryos turn, fuse the heart primordia, close the neural tube, begin overt organogenesis and start to grow very rapidly. Neural and mesenchymal progenitor cells have central roles in many of these processes. Their massive death and reduced rate of proliferation in SoxC -null embryos are thus sufficient to account for the failure of these embryos to undergo organogenesis. Many distinct organs are affected in SoxC partial mutants, but failure to form or hypoplasia is a common feature. All defects could thus have the same origin, that is, a reduction in the number of progenitor cells. The high expression level of SoxC genes in neural and mesenchymal cells, and our observation that cell death also occurs when the genes are specifically inactivated in these cells, strongly suggests that SoxC genes function in a cell-autonomous manner. The demonstration that SoxC genes are necessary for neural and mesenchymal cell survival raises the question of whether they are master regulators. This appellation would require SoxC genes to be sufficient for cell self-renewal as well, including cell identity, survival and proliferation. This cannot be tested easily in early embryos, in which cell death is minimal andmaintaining cells at a progenitor stage would be as detrimental as losing them. However, the results of recent studies are consistent with master roles for SoxC proteins. For instance, overexpression of Sox4 in glial cells in transgenic mice was shown to be sufficient to maintain the cells at an early stage [43] , [44] . Silencing of SOX4 was shown to induce apoptosis of prostate cancer cells in vitro , whereas stable expression in non-transformed prostate cells enabled colony formation in soft agar, supporting the notion that SOX4 might be both needed and sufficient for cell self-renewal [24] . SoxC genes may thus be master regulators in neural and mesenchymal progenitors in the same way as Sox2 is a master regulator for embryonic stem cells, and as other Sox genes are master regulators in differentiated cell lineages. This supports the concept that Sox genes fulfil critical functions in all cell types, whether pluripotent, multipotent or unipotent. Essential roles in neural and mesenchymal cells do not exclude the possibility that SoxC genes also control cell fate in differentiated cell lineages later. Many Sox genes, including Sox2 , have indeed been shown to have distinct roles in more than one cell type, by cooperating with different partners in different cell types [45] . In fact, Sox4 was shown to promote B- and T-cell expansion and differentiation [15] , [16] ; Sox4 and Sox11 control pan-neuronal differentiation in the central nervous system [19] , and Sox4 +/− mice develop osteopenia in adulthood, possibly because of defects in osteoblast proliferation, differentiation and mineralization [18] . At present, the only gene that has been convincingly demonstrated to be a SoxC direct target is Tubb3 [19] . It was validated through expression changes in vivo and in vitro , and through DNA-binding and transactivation assays in vitro . However, chromatin immunoprecipitation data were not provided to definitively demonstrate that SoxC proteins bind Tubb3 in live cells. Other studies proposed additional SoxC targets on the basis of expression changes on SoxC knockdown or overexpression in vitro , and on the basis of Sox consensus sites in promoter regions, but these studies lacked in vivo validation [46] . Our search for SoxC targets led to Tead2 . We showed that Tead2 expression closely matches SoxC expression in wild-type embryos and is significantly downregulated in SoxC mutant embryos and cultured cells. SoxC proteins also bind Tead2 in vivo through conserved elements in the promoter and first intron, and these sites are necessary for SoxC-dependent transactivation of reporter genes. Furthermore, we showed that Tead2 functionally interacts with SoxC genes in vivo and that expression of a constitutively active form of Tead2 is sufficient to prevent cell death on SoxC inactivation in vitro . These data thus identify Tead2 as one of the few direct targets of SoxC proteins currently known in neural cells and as a first one in mesenchymal cells. We selected Tead2 from a list of genes downregulated in SoxC mutant cells because of its implication as a transcriptional mediator of the Hippo signalling pathway. Similar to SoxC genes, this pathway is implicated in the intrinsic control of organ and cancer growth [36] . Moreover, Tead1/2 -null mice fail in development at the same time as SoxC mutants, with no impairment in embryo patterning and cell lineage specification, but with decreased cell survival and proliferation. Of the four Tead genes, however, only Tead2 expression was downregulated in SoxC mutants. Together with the fact that Tead2 -null mice are not as severely affected as SoxC mutants [37] , these data imply that SoxC proteins, similar to master genes, must control other important genes that are yet to be identified. Our microarray screening revealed that the expression level of many other genes was altered in SoxC mutants. However, the relevance of their expression changes is unknown, as the functions of these genes remain elusive. The fact that only a constitutively active form of Tead2, and not the wild-type protein, was able to rescue the cell death fate of SoxC -null cells in vitro suggests that the cells did not have enough YAP/TAZ coactivator available in the nucleus to associate with exogenous Tead2. As YAP/TAZ are phosphorylated and subsequently degraded in the cytoplasm downstream of Hippo signalling, it is possible that SoxC proteins control more signalling components than Tead2 in the Hippo pathway to allow YAP/TAZ to translocate into the nucleus and activate gene transcription in cooperation with Tead2. Our microarray screening experiment did not reveal gene expression changes for other Hippo signalling components, but it is possible that some of these components remain unknown or that SoxC proteins control protein activity rather than the gene expression of other Hippo signalling components. Neural and mesenchymal progenitor cells have important roles beyond development in adult tissue homeostasis and repair, and in such diseases as cancers. The same is certainly true for SoxC genes, the upregulation and likely involvement of which in various types of cancers have been profusely documented. It is thus anticipated that the results of this study will inspire and help future studies to further elucidate the molecular control of embryonic neural and mesenchymal progenitors, the molecular control of neural and mesenchymal adult stem cells and the functions of SoxC genes in these cells. Mice Mouse Sox11 and Sox12 conditional null alleles were obtained by flanking the gene coding sequences with loxP sites ( Supplementary Figs. S1 and S2 ). Targeting vectors were constructed using SvEv129 genomic DNA. The frt-neo r -frt-loxP neomycin-resistance cassette [47] and MC1tkpA thymidine kinase cassette [48] were previously described. Routine genotyping of mice was carried out by PCR. Sox11 + and Sox11 fl+ allele-specific segments were amplified using the primers FPA (TTCGTGATTGCAACAAAGGCGGAG) and RPA (GCTCCCTGCAGTTTAAGAAATCGG). A Sox11 fl− allele-specific segment was amplified using primers FPB (AGAGAGCGAGAAATCAAGCGAGTG) and RPB (CTGCCGACGTCTTTCAGACTTCAA). For the Sox12 + allele, the primers were FPA (CCTTCTTGCGCATGCTTGATGCTT) and RP (GGAAATCAAGTTTCCGGCGACCAA), and for the Sox12 − allele, the primers were FPB (ATGCAAATGCTGAGTTCTCTGCCC) and RP. All PCR reactions were carried out in standard buffer supplemented with 2 mM MgCl 2 , with 35 cycles of 94 °C for 15 s, 65 °C for 75 s and 72 °C for 90 s, followed by a final extension step at 72 °C for 7 min. PCR for Sox12 + and Sox12 − was carried out in standard buffer supplemented with 2.75 mM MgCl 2 and 5% dimethylsulphoxide, respectively. All other alleles and transgenes were previously described. Control and mutant mice were analysed as littermates on a 129xB6 hybrid genetic background. Whole-mount embryo procedures 5-bromo-4-chloro-3-indolyl-β- d -galactoside staining and skeletal preparations were performed as described [49] . Scanning electron microscopy was carried out following a standard procedure and embryos were analysed on a JOEL JSM 5310 scanning electron microscope using JOEL Orion image acquisition and handling controls. RNA in situ hybridization was carried out using digoxygenin-labelled riboprobes. Embryos were fixed for 2 h in 2% paraformaldehyde in 0.1% Tween-20 in PBS (PBST), digested for 10 min with 10 μg ml −1 proteinase-K in PBST and postfixed for 20 min in 2% paraformaldehyde in PBST. Prehybridization was performed for 6 h at 65 °C before adding 1 μg ml −1 of probe and hybridizing for 18–24 h. After posthybridization washes, embryos were blocked in 20% decomplemented goat serum, 2% BM-blocking reagent (Roche) in 0.1 M maleic acid, pH 7.5, 0.15 M NaCl, 0.1% Tween-20 for 3 h, and then probed with a 1/2,000 dilution of alkaline phosphatase-conjugated antidigoxygenin antibody (Roche) for 18–24 h at 4 °C. For chromogenic detection, embryos were incubated in 250 μg ml −1 nitroblue tetrazolium and 125 mM 5-bromo-4-chloro-3-indolyl phosphate. The reaction was stopped by washing abundantly with 10 mM Tris-HCl pH7.5, 0.15 M NaCl, 0.1% Tween-20. Procedures on paraffin sections Whole embryos or specific organs were fixed in 4% paraformaldehyde in PBS for at least 12 h at 4 °C, dehydrated, embedded in paraffin, cut into 7 μm-thick sections and stained either with haematoxylin and eosin Y or with Alcian blue and nuclear fast red. RNA in situ hybridization of paraffin-embedded embryo sections was carried out using [ 35 S]-rUTP-labelled RNA probes as described [50] . Procedures on frozen sections For BrdU analysis of cell proliferation, pregnant dams were injected intraperitoneally with BrdU solution (Invitrogen, # 00-0103) at 0.1 ml g −1 of body weight 45 min before being killed. Embryos were fixed for 20 min in 4% paraformaldehyde in PBS and embedded in OCT medium (Sakura Technologies). Cryosections of 10 μm thickness were obtained. TdT-mediated dUTP nick end labeling assay was performed using the ApopTag kit (Chemicon, S7010). For immunostaining, sections were incubated with 0.5 μg ml −1 anti-BrdU FITC-conjugated antibody (BD Bioscience) or antiphospho-histone-3 Ser10 rabbit polyclonal antibodies (Cell Signaling Technologies) for 18 h at 4 °C. AlexaFluor 488-conjugated anti-rabbit antibody (Invitrogen) was used as secondary antibody for phospho-histone-3 immunodetection. Sections were mounted in DAPI-containing Vectashield medium (Vector Labs). Image acquisition Embryos were photographed using a Nikon SMZ1500 microscope equipped with C-W10_20 lenses and a Spot Insight digital camera. Sections were analysed with an Olympus BX50 microscope equipped with Olympus Uplanapo ×10, 0.40-numerical aperture and Olympus Uplanapo 20×, 0.70-numerical aperture infinity-corrected (effective numerical aperture, 0.17) lenses. Images were captured with a Polaroid DMC2 digital camera. Primary culture and adenovirus infection of limb bud cells Limb buds from E11.5 embryos were dissociated in 0.25% trypsin-EDTA for 10 min at 37 °C. Cells were passed through a 40 μm nylon cell strainer and cultured in DMEM containing 10% FCS. Sox4 and Sox11 were inactivated by treating limb bud cells with 100 plaque-forming unit per cell Cre recombinase-expressing adenovirus (Iowa University) for 24 or 48 h. Control cells were infected with LacZ-expressing adenovirus (Iowa University). Transfection and adenovirus infection of osteoblasts Calvaria from 2-day-old Sox4 fl/fl 11 fl/fl 12 −/− mice were digested in 0.1 mg ml −1 collagenase P and 0.25% trypsin for 1 h at 37 °C. Cells were passed through a 40 μm nylon cell strainer and cultured for 48 h in MEM containing 10% FCS and then replated at 3×10 5 cells/10 cm 2 dish in the same medium, which keeps osteoblasts at a precursor stage [51] . After 16 h, mixtures of 500 ng of pLVX-Amcyan1-C1 vector (Clontech); 500 ng of Sox4 expression plasmid or pOZ retroviral vector encoding no protein, wild-type Tead2 or a Tead2/YAP fusion protein [39] ; and 3 μl of FuGENE6 (Roche) were added to the cells. After 12 h, cells were infected with AdeCre or AdelacZ. Apoptosis assay and cell-cycle analysis in cultured cells Cultured cells were collected by digestion with trypsin-EDTA, and 5×10 5 cells were used per assay. For the apoptosis assay, cells were fixed with 1% paraformaldehyde for 2 h, washed with PBS and further fixed for 16 h in 70% ethanol at −20 °C. TdT-mediated dUTP nick end labeling (assay) staining was carried out with an Apo-BrdU kit (BD-Pharmingen). For osteoblasts co-transfected with Amcyan and Tead2 or Sox4 expression plasmids, the percentage of cells undergoing apoptosis was measured according to the ratio of cells positive for Amcyan only and cells positive for both Amcyan and BrdU. For cycle analysis, cells were fixed for 16 h in 70% ethanol at −20 °C and washed with PBS. After incubation with 0.1 mg ml −1 RNase A at 37 °C for 15 min, cells were stained with 25 μg ml −1 propidium iodide. Fluorescence-activated cell sorting was carried out using an LSRII instrument (BD Biosciences), and data were analysed using FlowJo software (Ashland). RNA assays Gene expression profiles were obtained from E11.5 limb bud cells cultured for 24 h in the presence of adenovirus. Total RNA was prepared using TRIzol (Invitrogen), followed by RNeasy columns (Qiagen) and treatment with 1 U of DNase I (Invitrogen) per μg RNA. Complementary RNA was generated and hybridized to Illumina MouseRef-8 v2 expression bead chips, according to the manufacturer's instructions. Genes differentially expressed by at least 1.5-fold in three independent experiments were identified using BeadStudio software (version3.0 from Illumina). For quantitative real-time reverse transcription–PCR, cDNA was synthesized using a Superscript III first-strand cDNA synthesis kit (Invitrogen) and amplified with gene-specific primers ( Supplementary Table S3 ) using SYBR green PCR master mix (Applied biosystems) on an ABI PRISM 7900HT qPCR instrument(Applied Biosystems). PCR conditions were one cycle at 95 °C for 10 s, followed by 40 cycles of 95 °C for 5 s and 60 °C for 30 s. Relative mRNA levels were calculated using the 2 −DD C T method [52] . RNA probes Sox4 , Sox11 and Sox12 RNA probes were previously described [11] . The probes for Fgf8 [53] , Myf5 [54] , Shh [55] and for Tead1 , Tead3 and Tead4 [56] were as described. The Bmp4 probe was a 1 kb fragment encompassing 5′ UTR and 5′ coding sequences in mouse cDNA (NM_007554). The HoxB9 probe encompassed nucleotides 980–1447 in mouse cDNA (NM_008270). The Otx2 probe encompassed nucleotides 562–1620 in the cDNA (NM_144841). The Pax1 probe encompassed nucleotides 358–675 in mouse cDNA (NM_008780). The Pax7 probe encompassed nucleotides 434–754 in mouse cDNA (NM_011039). The Ptc1 probe was the entire mouse cDNA sequence (NM_008957). The Tead2 probe encompassed nucleotides 1,130–1,816 in mouse cDNA (GenBank NM_011565). Reporter assays Mouse Tead2 sequences were amplified from genomic DNA using PCR primers designed with Hin dIII sites at the 5′ end, and cloned into the promoterless pA3luc plasmid [54] . Point mutations in Sox-binding sites were introduced by Stratagene Quick change mutagenesis. FLAG-Sox expression plasmids were previously published [11] . For transient transfection, 3×10 5 Cos-1 and C3H-10T1/2 cells were plated per 10 cm 2 dish. Mixtures of 200 ng pSV2-betaGal plasmid, 200 ng Sox expression plasmid, 600 ng reporter plasmid and 3 μl FuGENE6 (Roche) were added to the cells 6 h after plating. Whole-cell extracts or chromatin was prepared 24 or 36 h later. Luciferase and β-galactosidase activities were assayed using the Dual-light combined reporter gene assay system (Applied Biosystems) and a Wallac victor 1,420 microplate reader (Perkin–Elmer). Reporter activities were normalized for transfection efficiency. Electrophoretic mobility shift assay This assay was performed as described [11] using double-stranded oligonucleotide probes. Sequences of the oligonucleotides used to generate probes are shown in Supplementary Table S4 . Chromatin immunoprecipitation Chromatin was prepared from C3H-10T1/2 cells transiently transfected with FLAG-Sox expression plasmids [57] . Briefly, 3×10 6 cells were crosslinked with 0.5% formaldehyde for 10 min, followed by addition of glycine at 125 mM. Chromatin was sheared by sonication to fragments averaging 400 bp in buffer containing 1% SDS, 10 mM EDTA, 50 mM Tris-HCl, pH 8.1 and protease inhibitor cocktail (Sigma). Chromatin containing 20 μg DNA was precleared with 15 μl protein G-coupled Dynal magnetic beads (Invitrogen), followed by immunoprecipitation with 4 μg anti-FLAG M2 antibody (Sigma) coupled to 15 μl protein G-coupled Dynal magnetic beads per experimental condition. Non-immune mouse IgG (Sigma) and monoclonal anti-RNA polymerase II antibody (Upstate) were used as controls. ATAACCACCTTCTCTCCTAGGGACC and TTGCCGGGAGCTTTGTTTGGGAAA primers were used to amplify the Tead2 PE1 region. AGATTAGAGATGTCCGTCTG and CTCCAATTTTGGACTCTTGA primers were used to amplify the Tead2 InS region. Col2a1 enhancer primers were as described [58] . PCR was carried out with one cycle at 94 °C for 3 min; 35 cycles at 94 °C for 30 s, 57 °C for 1 min and 72 °C for 1 min; and one cycle at 72 °C for 5 min. How to cite this article: Bhattaram, P. et al . Organogenesis relies on SoxC transcription factors for the survival of neural and mesenchymal progenitors. Nat. Commun. 1:9 doi: 10.1038/ncomms1008 (2010). Copyright: © 2010 Bhattaram, P. et al. This is an open-access article distributed under the terms of the Creative Commons Attribution License, which permits unrestricted use, distribution and reproduction in any medium, provided the original author and source are credited.